The sharp structural switch of covalent cages mediated by subtle variation of directing groups 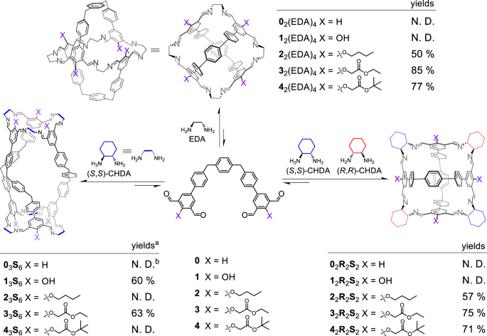Fig. 1: Structural formulae and NMR yields of a series of cage products including 22R2S2, 32R2S2, 42R2S2, 03S6, 13S6, 33S6, 22(EDA)4, 32(EDA)4, 42(EDA)4. These cages are produced by condensing each of the corresponding tetraformyl precursors including0-4, and the bisamino partner namely racemictrans-CHDA, (S,S)-CHDA, or EDA.aThe yields are all determined by using internal standard in the corresponding1H NMR samples without isolating the corresponding products.bN. D. means Not Determined, because either the target molecules were not produced with observable yields, or the products are generated within a library of mixture whose1H NMR spectrum is too complicated to determine the corresponding yields. It is considered a more formidable task to precisely control the self-assembled products containing purely covalent components, due to a lack of intrinsic templates such as transition metals to suppress entropy loss during self-assembly. Here, we attempt to tackle this challenge by using directing groups. That is, the self-assembly products of condensing a 1:2 mixture of a tetraformyl and a biamine can be precisely controlled by slightly changing the substituent groups in the aldehyde precursor. This is because different directing groups provide hydrogen bonds with different modes to the adjacent imine units, so that the building blocks are endowed with totally different conformations. Each conformation favors the formation of a specific product that is thus produced selectively, including chiral and achiral cages. These results of using a specific directing group to favor a target product pave the way for accomplishing atom economy in synthesizing purely covalent molecules without relying on toxic transition metal templates. Mother Nature avoids byproducts in synthesis by taking advantage of reversible bonding forces [1] , [2] , [3] , [4] . The reversible nature of these supramolecular interactions allows synthetic errors to be checked and corrected. This biological capability inspires chemists to employ either noncovalent forces [5] , [6] , [7] or dynamic bonds [8] , [9] , [10] , [11] , [12] , [13] , [14] as the reaction motifs in synthesizing artificial systems. Henceforth, high-yielding syntheses could be accomplished without relying on tedious stepwise procedures, by sophisticatedly designing and tuning the geometries and conformations of the building blocks that allows the corresponding target products to represent the thermodynamic minima in self-assembly. One of the most successfully developed reversible reactions is metal-ligand coordination [15] , [16] , [17] , [18] , [19] , [20] , [21] , [22] , [23] , [24] , [25] , [26] , [27] , [28] . A variety of molecules with complex architectures and topologies have been successfully self-assembled [29] , [30] , [31] , [32] , [33] , [34] , some of which [16] , [17] , [21] , [22] , [23] , [30] were obtained in close to quantitative yields. Here, transition metal cations with fixed coordination modes are able to dictate the corresponding organic ligands to orientate in specific manners that favor the formation of some specific products. Subtle changes of the organic ligands in geometry and/or size might lead to dramatic variation in self-assembly pathway [35] , [36] , [37] , [38] , [39] , [40] , [41] , [42] . The same level of success, however, has not been achieved in the systems containing purely covalent components that are often relatively more flexible, in which the intrinsic templates namely transition metals are absent. The implication is that, the self-assembled products via dynamic covalent chemistry [8] , [9] , [10] , [11] , [12] , [13] , [14] , [43] , [44] , [45] such as imine formation [46] , [47] , [48] , [49] , [50] , [51] , [52] , [53] , [54] , [55] , [56] , [57] are thus often less controllable compared to the coordinative counterparts, despite a few exceptions [56] , [58] , [59] , [60] , [61] , [62] , [63] . For example, Cooper [64] et al. demonstrated that the amino precursors containing odd or even numbers of methylene units favored the formation of [2 + 3] or [4 + 6] cages, respectively. Mastalerz [13] et al. discovered that an organic cage self-assembled via boronic ester bond formation could undergo dimerization and form a catenane in solid-state, when switching the constitution of the side chains in the tetraol precursor. More recently, the same group [65] indicated that introducing methoxy or thiomethyl unit onto the framework of an imine cube led to occurrence of dimerization and trimerization, forming catenanes in solution. Mukherjee [66] et al. employed intramolecular hydrogen bonding to direct self-sorting. The group led by Beuerle [67] obtained a highly strained organic cage whose formation would be otherwise unlikely to occur without intramolecular driving forces namely hydrogen bonds. In the present work, we employed directing groups to precisely control the self-assembly products based on imine formation. These directing groups mediate or determine the conformations of the building blocks, by providing hydrogen bonds with different modes to the latter. Each of these preorganized conformations of the building blocks favors one specific cage compound that is produced as the predominant product. To be more specific, a pseudo-linear tetraformyl precursor containing two isophthalaldehyde units and trans -cyclohexane-1,2-diamine ( trans -CHDA), which is either enantiomerically pure or the racemic mixture, are combined for self-assembly. Subtle variation in the substituents located in each isophthalaldehyde residue switches the self-assembly products between two types of constitutionally different cage molecules, including a [3 + 6] chiral cage and a [2 + 4] achiral cage. In the case of OH unit whose acid proton acts as a hydrogen bond donor, intramolecular hydrogen bonds drive the two formyls and/or the resultant imine units on both sides to orientate in an exo - endo conformation. Such conformation favors the production of a [3 + 6] chiral cage, which is composed of three equivalents of the tetraformyl precursor and six equivalents of enantiomerically pure trans -CHDA. When the racemic trans -CHDA is used in self-assembly, narcissistic self-sorting occurs, generating a pair of enantiomers of the [3 + 6] chiral cage each containing only one type of enantiomer of trans -CHDA. As a comparison, an alkoxy substituent containing no acidic protons affords the two formyls and/or imines an exo - exo conformation [68] . When the tetraformyl precursor is combined with the racemic mixture of trans -CHDA in a 1:2 ratio, a meso [2 + 4] cage is produced as the only observable product, which is composed of two equivalents of the tetraformyl precursor and four equivalents of racemic trans -CHDA. More interestingly, when the substituent is an ester unit containing protons with modest acidity, both exo - endo and exo - exo conformations become thermodynamically feasible. The self-assembled products are then determined by the chirality of the bisamine precursors. That is, enantiomerically pure and racemic bisamine favor the [3 + 6] and [2 + 4] products, respectively. Physicochemical analysis based on NMR spectroscopic results, solid-state structures, as well as theoretical calculation results indicated that these self-assembly preferences stem from the self-assembly products attempting to minimize intramolecular steric hindrance, by keeping all the imine protons in the syn conformation [69] , [70] relative to the corresponding adjacent methine proton in the cyclohexyl unit. Each of the five structurally analogous tetraaldehyde precursors 0 - 4 (Fig. 1 ), whose synthetic procedures are described in the Supplementary Information (Supplementary Figs. 5 , 7 , 9 , 11 and 14 ), contains two isophthalaldehyde units. The differences between these five precursors lie in the substituents grafted in each of the isophthalaldehyde moiety between the two formyl units (Fig. 1 ), which are ‒H ( 0 ), ‒OH ( 1 ), ‒OC 4 H 9 ( 2 ), ‒OCH 2 COOC 2 H 5 CH 3 ( 3 ), and ‒OCH 2 COOC(CH 3 ) 3 ( 4 ), respectively. A pair of enantiomers of a chiral bisamine, namely (1 S ,2 S )-cyclohexane-1,2-diamine (( S , S )-CHDA) and (1 R ,2 R )-cyclohexane-1,2-diamine (( R , R )-CHDA), as well as ethylenediamine (EDA) were used as the amino partners for self-assembly (Fig. 1 ). Fig. 1: Structural formulae and NMR yields of a series of cage products including 2 2 R 2 S 2 , 3 2 R 2 S 2 , 4 2 R 2 S 2 , 0 3 S 6 , 1 3 S 6 , 3 3 S 6 , 2 2 (EDA) 4 , 3 2 (EDA) 4 , 4 2 (EDA) 4 . These cages are produced by condensing each of the corresponding tetraformyl precursors including 0 - 4 , and the bisamino partner namely racemic trans -CHDA, ( S,S )-CHDA, or EDA. a The yields are all determined by using internal standard in the corresponding 1 H NMR samples without isolating the corresponding products. b N. D. means Not Determined, because either the target molecules were not produced with observable yields, or the products are generated within a library of mixture whose 1 H NMR spectrum is too complicated to determine the corresponding yields. Full size image We first combined 1 (2.5 mM) and ( S , S )-CHDA (Fig. 2A ) in a 1:2 ratio in CDCl 3 . After heating the solution at 50 °C for 6 h, the 1 H NMR spectrum (Fig. 2B ) was recorded, in which a set of sharp resonances were observed, indicating a product with a symmetrical structure was obtained as the predominant product. Mass spectrum (Supplementary Fig. 28 ) indicated that this product is a [3 + 6] product, namely composed of three equivalents of 1 and six equivalents of ( S , S )-CHDA. This product is referred to as 1 3 S 6 . In the 1 H NMR spectrum (Fig. 2B ), each of the resonances corresponding to the protons in the isophthalaldehyde residues, including both the imine e / e’ and the phenyl c / c’ , splits into two peaks. This observation indicated that in each isophthalaldehyde residue, the two imine units have two different orientations, namely either exo or endo with respect to the central OH group (Fig. 3B , middle). The framework of 1 3 S 6 is chiral, resulting from the stereo chirality of the ( S , S )-CHDA precursor. The chirality of 1 3 S 6 was supported by 1 H NMR spectrum (Supplementary Fig. 29 ) in which the two protons in the methylene f become diastereotopic. The solid-state sample of 1 3 S 6 was obtained by adding MeOH into its solution in chloroform and collecting the precipitate via filtration. The solid of 1 3 S 6 was re-dissolved in CDCl 3 , whose 1 H NMR spectrum was essentially the same as the before precipitation, indicated that 1 3 S 6 was rather kinetically inert and did not undergo observable degradation during precipitation and re-dissolving. In the 1 H NMR spectrum (Fig. 2B ) of 1 3 S 6 , a few small broad resonances were observed, indicating that some oligomeric or polymeric byproducts were also generated. These broad resonances were not removed, even after we attempted to purify 1 3 S 6 via precipitation. We thus used NMR yield to quantify the production of each cage in this article, by adding an internal standard in the NMR sample. The self-assembly yield of 1 3 S 6 was determined to be 60% (Supplementary Fig. 76 ). The cage 1 3 R 6 , which is the enantiomer of 1 3 S 6 , was also self-assembled in a similar procedure (Supplementary Fig. 16C ), by condensing 1 and ( R , R )-CHDA in CDCl 3 . The circular dichroism (CD) spectra (Supplementary Fig. 33B ) of both 1 3 S 6 and 1 3 R 6 were recorded, showing mirror-like images. When 1 was combined with a racemic mixture of ( R , R )-CHDA and ( S , S )-CHDA in CDCl 3 , narcissistic self-sorting [71] , [72] , [73] occurred (Supplementary Fig. 17 ), yielding a racemic mixture of 1 3 S 6 and 1 3 R 6 as the major product. Fig. 2: The self-assembly of a pair of cage enantiomers 1 3 S 6 and 1 3 R 6 . ( A ) Structural formulae of 1 3 S 6 and 1 3 R 6 by condensing the precursor 1 and the corresponding bisamino partners namely either ( S , S )-CHDA or ( R , R )-CHDA. Narcissistic self-sorting occurs when 1 is combined with the racemic mixture of ( S , S )-CHDA and ( R , R )-CHDA. ( B ) Partial 1 H NMR spectrum (600 MHz, CDCl 3 , 298 K) of 1 3 S 6 . Some of the key resonances are labeled, which were assigned based on the corresponding two-dimensional NMR spectra shown in Supplementary Figs. 31 and 32 . The full spectrum is also shown in Supplementary Fig. 29 . ( C ) Solid-state structures of 1 3 S 6 obtained from single-crystal X-ray diffraction analysis. Oxygen atoms, red; nitrogen, blue; carbon, gray. Hydrogen atoms and disordered solvent molecules are omitted for clarity. We also expanded the terminal part of the cage 1 3 S 6 for the sake of clarity. It is clearly observed that all the imine protons adopt the syn conformation relative to the corresponding methine protons, as labeled with red double-head arrows. Two intramolecular hydrogen bonds between the central OH proton and the imine nitrogen on one side, and the central OH oxygen and the imine proton on the other side, are labeled with black dashed lines. Full size image Fig. 3: The possible conformations of the imine adducts of isophthalaldehyde derivatives bearing different central substituents between the two imine units. These different central substituents include ( A ) H, ( B ) OH, ( C ) alkoxy (OR) unit, and ( D ) ester (OCH 2 COOC 2 H 5 ) chain. Hydrogen bonding interactions occurs between the central substituents and the two imine units on both sides, which are marked with red dashed lines. OH favors the exo-endo conformation, while the OR unit favors exo-exo one. In the case of the ester, both exo-exo and exo-endo are stable conformations, driven by hydrogen bonding with different modes. These relatively stable conformations are encircled with red rectangles. ( E ) Two conformations of an imine compound, including syn (right) and anti (left). The syn conformer is more favored than the anti one due to smaller steric hindrance in the former conformer. Full size image Single crystals of the cage 1 3 S 6 (Fig. 2C ), as well as the racemic mixture (Supplementary Fig. 88 ) of 1 3 S 6 and 1 3 R 6 , were obtained by vapor diffusion of methanol or acetonitrile into the corresponding solutions in CHCl 3 or DMF, respectively. The solid-state structures of both 1 3 S 6 and 1 3 R 6 convinced the exo - endo conformation of the two imine units in each isophthalaldehyde residue, consistent with the 1 H NMR spectroscopic results. This exo - endo conformation is favored by the formation of intramolecular hydrogen bonds (Fig. 3B , middle), namely that the oxygen atom in the central OH forms hydrogen bond with the imine proton on one side, while the OH proton forms hydrogen bond with the imine nitrogen atom on the other side. These two types of hydrogen bonds are clearly observed in the solid-state structures (Fig. 2C , black dashed lines). Such exo - endo conformation was also observed in many cage systems containing trans -CHDA [61] , [74] , [75] , [76] . The exo - endo conformation allows all the imine protons to orientate in a syn conformation relative to the corresponding adjacent methine protons (Fig. 2C , red double-head arrows). According to a report by Gawronski [70] , such syn conformer is thermodynamically more favored than the anti counterpart by 0.92 kcal/mol, due to larger steric hindrance in the latter conformer (Fig. 3E ). We also combined 1 and EDA, which is a less preorganized counterpart of trans -CHDA. Heating the mixture in CDCl 3 led to the generation of a library of oligomeric and polymeric precipitates, instead of a putative [3 + 6] cage namely 1 3 (EDA) 6 . Such results indicate that conformation preorganization is also of importance in the bisamino precursors. In order to strengthen our proposition that the OH group in 1 plays a predominant role in favoring the formation of the corresponding [3 + 6] cages namely either 1 3 S 6 or 1 3 R 6 , we synthesized three analogs including 0, 2 as well as 3 , in which the central OH substituents in 1 are replaced by other units namely H, alkyloxy and ester respectively. The precursor 0 can be considered as a counterpart of 1 without any directing groups. 0 and ( S , S )-CHDA were combined in CDCl 3 in a 1:2 ratio. After heating the corresponding solution at 50 °C for 4 h, the 1 H NMR spectrum (Supplementary Fig. 23A ) indicated that an analog of 1 3 S 6 , namely 0 3 S 6 was produced as the major product, accompanied with a [2 + 4] product 0 2 S 4 as a kinetic product. The formation of both 0 3 S 6 and 0 2 S 4 was convinced by mass spectrometry (Supplementary Fig. 24 ). Further heating the reaction mixture for 120 h converted most 0 2 S 4 into 0 3 S 6 , as inferred from the observation that the molecular ion peak corresponding to the [2 + 4] product weakened significantly (Supplementary Fig. 25 ). Even heating the solution for no less than 120 h, the resonances corresponding to 0 2 S 4 with small intensity were still observable in the 1 H NMR spectrum (Supplementary Fig. 23C ), indicating that the conversion from 0 2 S 4 into 0 3 S 6 was not complete. The NMR yield of 0 3 S 6 was determined to be 70% (Supplementary Fig. 84 ). Compared to 1 , the precursor 0 is lack of the OH directing group, so that the 0 3 S 6 is thermodynamically less favored. Combining 0 and the racemic CHDA in a 1:2 ratio also produced the racemic mixture of 0 3 S 6 and 0 3 R 6 as major products. However, this narcissistic self-sorting was much less successful compared to the aforementioned system involving 1 , i.e., more oligomeric or polymeric byproducts (Supplementary Fig. 27 ) were observed in the corresponding 1 H NMR spectrum. We then combined either 2 or 3 (2.5 mM) with a racemic mixture of trans -CHDA in a 1:2 ratio in CDCl 3 . After heating at 50 °C for 6 h, the 1 H NMR spectra (Fig. 4B and Supplementary Fig. 48 ) and mass spectra (Supplementary Figs. 34 and 47 ) of both solutions were recorded. Mass spectrum indicated that in both cases, [2 + 4] products were generated. That is, each product is composed of two equivalents of tetraformyl precursors (i.e., 2 or 3 ) and four equivalents of trans -CHDA, namely either ( S , S )-CHDA or ( R , R )-CHDA. Fig. 4: The self-assembly of a series of achiral cages, including 2 2 R 2 S 2 , 3 2 R 2 S 2 and 4 2 R 2 S 2 . ( A ) Structural formulae of the cages 2 2 R 2 S 2 , 3 2 R 2 S 2 and 4 2 R 2 S 2 , by condensing a 2:1 mixture of racemic trans -CHDA and the corresponding tetraformyl precursor namely 2, 3 and 4 , respectively. ( B ) Partial 1 H NMR spectrum (600 MHz, CDCl 3 , 298 K) of 2 2 R 2 S 2 . Some of the key resonances are labeled, which were assigned based on the corresponding two-dimensional NMR spectra shown in the Supplementary Figs. 37 and 38 . The full spectrum is shown in the Supplementary Fig. 35 . Solid-state structures of 2 2 R 2 S 2 including ( C ) side view) and ( D ) top view, as well as 3 2 R 2 S 2 including ( E ) side view) and ( F ) top view, which were obtained from single-crystal X-ray diffraction analysis. Oxygen atoms, red; nitrogen, blue; carbon, gray. Hydrogen atoms and disordered solvent molecules are omitted for clarity. Full size image Single crystals of these two self-assembled products were obtained by vapor diffusion of either methanol or diethyl ether into the corresponding solutions in CHCl 3 , respectively. The solid-state structures unambiguously indicated that two cage products, namely 2 2 R 2 S 2 and 3 2 R 2 S 2 were obtained (Fig. 4 C–F). In the framework of both 2 2 R 2 S 2 and 3 2 R 2 S 2 , the two imine bonds in each of the isophthalaldehyde residues orientate in an exo - exo manner. This conformation is in sharp contrast to the exo - endo conformation in the case of either 1 3 S 6 or 1 3 R 6 containing OH substituents. The exo - exo conformation is favored by the formation of intramolecular five-member ring hydrogen bonds between the central oxygen atom and the two imine protons on both sides (Fig. 3C , left), assisted by the repulsion between the central oxygen and two imine nitrogen atoms. In the framework of either 2 2 R 2 S 2 or 3 2 R 2 S 2 , the four trans -CHDA residues distribute in an RSRS manner. That is, each isophthalaldehyde residue is connected by two different enantiomers of trans -CHDA. Such ligand distribution affords each cage namely either 2 2 R 2 S 2 or 3 2 R 2 S 2 two plane symmetries, affording both 2 2 R 2 S 2 and 3 2 R 2 S 2 meso structures. In addition, as expected, each imine proton adopts the more favored syn conformation with respect to the corresponding axial methine proton. The 1 H NMR spectra (Fig. 4B and Supplementary Fig. 48 ) of both 2 2 R 2 S 2 and 3 2 R 2 S 2 are similar. In the 1 H NMR spectrum (Fig. 4B ) of 2 2 R 2 S 2 , a few singlets corresponding to the protons including e , c and g are observed. The simple patterns of both 1 H NMR spectra convince that both 2 2 R 2 S 2 and 3 2 R 2 S 2 are highly symmetrical, consistent with the corresponding solid-state structure. It is noteworthy that because both ( R , R )-CHDA and ( S , S )-CHDA are involved in self-assembly, the cage containing four trans -CHDA residues has theoretically nine stereoisomers. However, the 1 H NMR spectra unambiguously indicates that only the RSRS ones, namely 2 2 R 2 S 2 or 3 2 R 2 S 2 , is produced selectively. This is because the RSRS isomer is the only one that can allow all the imine protons to adopt the more favored syn conformation with respect to corresponding axial methine protons. This unlikely occurring social self-sorting behavior was also reported by Mastalerz recently [77] . Both 2 2 R 2 S 2 and 3 2 R 2 S 2 were isolated as solid-state compounds by adding MeOH into the corresponding solutions in chloroform and collecting the precipitates via filtration. Again, NMR yields were used to quantify their production, given that oligomeric or polymeric impurities rendered the isolated yields less accurate. By using internal standard in the corresponding NMR samples, the yields (Supplementary Figs. 77 and 79 ) of 2 2 R 2 S 2 and 3 2 R 2 S 2 were determined to be 57% and 75%, respectively. We also combined either 2 or 3 (2.5 mM) with EDA (5.0 mM) in CDCl 3 , yielding two self-assembled products whose 1 H NMR spectra (Supplementary Figs. 43 and 53 ) are very similar as those of 2 2 R 2 S 2 and 3 2 R 2 S 2 . Mass spectra (Supplementary Figs. 42 and 52 ) confirmed that two cages namely 2 2 (EDA) 4 and 3 2 (EDA) 4 were self-assembled, whose yields (Supplementary Figs. 78 and 80 ) are 50 % and 85 %, respectively. It is still unclear why the yields of 3 2 R 2 S 2 and 3 2 (EDA) 4 are higher compared to 2 2 R 2 S 2 and 2 2 (EDA) 4 . We hypothesize that the precursor 3 contains two ester side chains. The protons in the methylene units that are connected directly by the ester oxygen atoms are more acidic compared to the methylene protons in 2 . The former protons form stronger CH-π interactions with the phenyl units in the cage framework. When the racemic trans -CHDA was replaced by enantiomeric pure ( S,S )-CHDA, self-assembly yielded totally different products. Heating a 1:2 mixture of 2 (2.5 mM) and ( S,S )-CHDA in CDCl 3 produced a library of mixture, whose 1 H NMR spectrum (Supplementary Fig. 19B ) showed a set of irregular resonances. Such observation indicated that the putative chiral cage namely 2 2 S 4 is not a thermodynamically favored product. The putative cage 2 2 S 4 can be considered as a chiral counterpart of 2 2 R 2 S 2 , in which two ( R,R )-CHDA residues are replaced by two ( S,S )-CHDA residues. However, in 2 2 S 4 , four of the eight imine protons adopt the thermodynamically disfavored anti conformation (Supplementary Fig. 19 ) with respect to the adjacent methine protons, making its formation less favored. Another putative product, namely 2 3 S 6 , an analog of 1 3 S 6 , was not observed in either 1 H NMR spectrum or mass spectrum. This is not surprising, given that the [3 + 6] products require the exo - endo conformation, while the alkyloxy directing groups in 2 , favor the exo - exo conformation in contrast. To our surprise, combining the tetraaldehyde 3 (2.5 mM) and ( S,S )-CHDA in CDCl 3 in a 1:2 ratio yielded a product whose 1 HNMR spectrum (Fig. 5B ) was in reminiscence of the aforementioned [3 + 6] product namely 1 3 S 6 . Mass spectrum (Supplementary Fig. 57 ) confirms that a chiral cage 3 3 S 6 was self-assembled as the predominant product, whose yield was determined to be 63 % (Supplementary Fig. 81 ). As occurred in 1 3 S 6 , the resonances corresponding to two imine protons in 3 3 S 6 also split into two peaks (Fig. 5B ), indicating that the two imines within each isophthalaldehyde residue adopt an exo - endo conformation. The exo - endo conformation was also supported by the NOESY spectrum (Supplementary Fig. 61 ) of 3 3 S 6 . That is, while the endo imine proton e’ undergoes coupling with one phenyl proton c’ in the isophthalaldehyde residue, the exo imine proton e undergoes coupling with the CH 2 proton k in the central side chain. The exo-endo conformation in the case of 3 3 S 6 was also driven by the formation of two different types of hydrogen bonds (Fig. 3D , middle). That is, one hydrogen bond forms between exo imine proton e and the central oxygen atom, while the second one forms between the endo imine nitrogen atom and the proton in the methylene unit h / h’ in ethyl unit of the ester. The occurrence of the latter hydrogen bonding results from the electron-withdrawing inductive effect of the ester oxygen atom, which renders the protons h / h’ relatively acidic. Such relatively acidic protons are absent in the case of 2 containing n -butoxy chains. It is therefore not surprising that 2 did not form the putative cage 2 3 S 6 . The occurrence of CH‒N hydrogen bonding forces in 3 3 S 6 is supported by its 1 HNMR spectrum (Fig. 5B ), in which the resonances corresponding to the methylene unit h / h’ in the ester split into two peaks, while the methylene unit k exhibits a singlet. In order to further strengthen our hypothesis that the acidic ester proton plays an important role in cage formation, we thus synthesized another tetraformyl precursor 4 (see its molecular formula in Fig. 1 ) containing tert -butyl acetate units. 4 contains ester functions while does not contain the protons with modest acidity as those in 3 . Combining 4 and ( S,S )-CHDA in a 1:2 ratio yielded a library of mixture (Supplementary Fig. 22 ), instead of 4 3 S 6 . This control experiment unambiguously supported our proposition that hydrogen bonding involving the ester side chains in 3 plays a critical role in favoring the formation of 3 3 S 6 . Addition of ( R,R )-CHDA into 3 3 S 6 gradually transformed latter into the [2 + 4] achiral cage 3 2 R 2 S 2 (Fig. 5A ). Furthermore, combining a mixture of pre-synthesized 3 3 S 6 and 3 3 R 6 with a 1:1 ratio also yielded the meso cage 3 2 R 2 S 2 . Apparently, the achiral cage 3 2 R 2 S 2 is more favored in terms of entropy compared with 3 3 S 6 , because the latter is composed of fewer building blocks compared to the former. 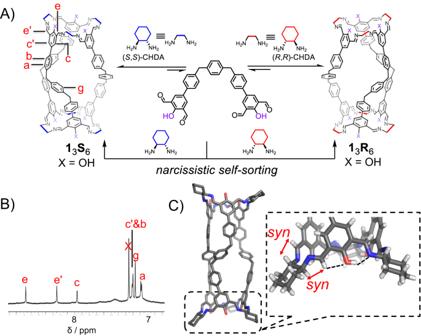Fig. 2: The self-assembly of a pair of cage enantiomers 13S6and 13R6. (A) Structural formulae of13S6and13R6by condensing the precursor1and the corresponding bisamino partners namely either (S,S)-CHDA or (R,R)-CHDA. Narcissistic self-sorting occurs when1is combined with the racemic mixture of (S,S)-CHDA and (R,R)-CHDA. (B) Partial1H NMR spectrum (600 MHz, CDCl3, 298 K) of13S6. Some of the key resonances are labeled, which were assigned based on the corresponding two-dimensional NMR spectra shown in Supplementary Figs.31and32. The full spectrum is also shown in Supplementary Fig.29. (C) Solid-state structures of13S6obtained from single-crystal X-ray diffraction analysis. Oxygen atoms, red; nitrogen, blue; carbon, gray. Hydrogen atoms and disordered solvent molecules are omitted for clarity. We also expanded the terminal part of the cage13S6for the sake of clarity. It is clearly observed that all the imine protons adopt thesynconformation relative to the corresponding methine protons, as labeled with red double-head arrows. Two intramolecular hydrogen bonds between the central OH proton and the imine nitrogen on one side, and the central OH oxygen and the imine proton on the other side, are labeled with black dashed lines. Fig. 5: The self-assembly of a chiral cage 3 3 S 6 that was transformed into 3 2 R 2 S 2 upon addition of ( R , R )-CHDA. ( A ) Structural formula of the cage 3 3 S 6 , by condensing a 2:1 mixture of ( S , S )-CHDA and 3 . Upon addition of ( R , R )-CHDA, 3 3 S 6 is converted into 3 2 R 2 S 2 . ( B ) Partial 1 H NMR spectrum (600 MHz, CDCl 3 , 298 K) of 3 3 S 6 . Some of the key resonances are labeled, which were assigned based on the corresponding two-dimensional NMR spectra shown in the Supplementary Figs. 60 and 61 . The full spectrum is shown in the Supplementary Fig. 58 . Full size image In order to confirm that the self-assembly preference results from the cage products attempting to keep all the imine protons in the syn conformation with respect to the corresponding methine protons, we further performed density functional theory (DFT) calculations at the BP86-D3/6-311G(d) level with the Gaussian 16 package [78] . Based on the solid-state structure of 2 2 R 2 S 2 obtained via crystallography, two putative cages, namely 2 2 S 4 and 2 2 S 2 R 2 , were optimized (see details in Supplementary Data 1 ). Here, 2 2 S 4 is a putative counterpart of 2 2 R 2 S 2 , whose two ( R,R )-CHDA residues are replaced with two ( S,S )-CHDA residues. 2 2 S 2 R 2 was obtained by replacing the two ( R,R )-CHDA and two ( S,S )-CHDA residues with ( S,S )-CHDA and ( R,R )-CHDA, respectively. In 2 2 R 2 S 2 , 2 2 S 4 and 2 2 S 2 R 2 , there are respectively zero, four and eight imine protons that adopt the less favored anti conformation with respect to the corresponding methine protons. The theoretical results revealed that the free energies of 2 2 S 4 and 2 2 S 2 R 2 are 5.4 kcal/mol and 9.1 kcal/mol with respect to that of 2 2 R 2 S 2 , respectively (Fig. 6 ). This confirms that the syn conformer is thermodynamically more favored than the anti counterpart in the cage framework. 2 2 R 2 S 2 , with all the imine protons in the syn conformation, is the most stable and favored product, which is fully consistent with our experimental results. Similar approaches were also used to calculate the free energies of 1 3 S 6 and a putative cage 1 3 R 6 ( anti ) (Supplementary Fig. 89 ). It is noteworthy that 1 3 S 6 and 1 3 R 6 ( anti ) are not a pair of enantiomers. The putative cage 1 3 R 6 ( anti ) was obtained by replacing all ( S,S )-CHDA residues in 1 3 S 6 with ( R,R )-CHDA, while keeping the conformations of all the imine bonds (details see Supplementary Data 1 ). In the putative cage 1 3 R 6 ( anti ), all imine protons adopt the anti conformation with respect to the adjacent methine protons. The calculations revealed that the free energy of 1 3 R 6 ( anti ) is 37.4 kcal/mol higher than that of 1 3 S 6 (Supplementary Fig. 89 ). Fig. 6: The optimized structures (top) and the structural formula (bottom) of 2 2 R 2 S 2 and its two putative less stable counterparts 2 2 S 4 and 2 2 S 2 R 2 , with their corresponding relative free energies. The calculation was performed by using DFT calculations at the level of BP86-D3 functional and 6-311 G(d) basis set. Full size image In summary, an ingenious approach to precisely control the self-assembly product based on imine condensation is developed, by introducing different directing groups to favor specific target products. When a tetraformyl precursor containing two isophthalaldehyde units and trans -CHDA are combined, the self-assembly products are very sensitive to the variation of the central substituents located in each isophthalaldehyde residue between two imine units. This is because the central directing groups provide hydrogen bonding with different modes to imine building blocks located on both sides. These intramolecular forces endow the imine units with specific conformations, each resembling and favoring a specific cage product that is produced selectively. To be specific, in the case of OH substituent group whose proton is rather acidic, the two imine bonds are preorganized in an exo - endo conformation, driven by two different hydrogen bonds in the form of either CH‒O or OH‒N. Such conformation favors the formation of a chiral [3 + 6] cage containing enantiomeric pure trans -CHDA residues. When the substituent group contains no acidic protons such as an alkoxyl unit, the two imine bonds have an exo - exo conformation driven by two identical hydrogen bonds namely CH‒O. Such conformation favors the formation of achiral [2 + 4] cages containing racemic trans -CHDA building blocks as the predominant product, implying the occurrence of social self-sorting. In the case of ester substituent group containing protons with modest acidity, both the exo - endo and exo - exo conformations are thermodynamically feasible. As a consequence, the self-assembly products are surprisingly determined by the chirality of the trans -CHDA, namely that enantiomeric pure and racemic trans -CHDA favor the [3 + 6] and [2 + 4] products respectively. Such preference results from a tendency that the imine protons attempt to adopt the syn conformation relative to the adjacent axial methine protons in the CHDA residues, in order to minimize steric hindrance. Our fundamental understanding of precisely controlling the thermodynamic stability of a target product by using directing group to regulate the intramolecular forces, is thus significantly improved. Such results help us to rule out the reliance of cationic transition metal templates that might be highly toxic. Future research includes self-assembly of cage molecules with larger cavities and water-solubility, so that these self-assembled hosts are employed for applications in some more challenging arenas, such as mimicking enzyme [79] , [80] , [81] , [82] in artificial systems. Self-assembly of 1 3 S 6 A 1:2 mixture of 1 (2.77 mg, 0.005 mmol) and ( S,S )-CHDA (1.14 mg, 0.01 mmol) was combined and dissolved in CDCl 3 (2 mL). The corresponding reaction mixture was heated at 50 °C for 6 h. 1 3 S 6 was self-assembled as the major product in the corresponding 1 H NMR spectrum, without further manipulation. The solid-state sample of 1 3 S 6 was obtained by adding MeOH into its solution in chloroform and collecting the precipitate via filtration. However, it is unsuccessful to purify 1 3 S 6 via precipitation, accompanied by the generation of some oligomeric or polymeric byproducts. We thus used a NMR yield (60 %) to quantify the production of 1 3 S 6 , by adding an internal standard in the NMR sample. Self-assembly of 2 2 R 2 S 2 , 3 2 R 2 S 2 and 4 2 R 2 S 2 A 1:2 mixture of the corresponding tetraformyl precursor ( 2, 3 or 4 , 0.005 mmol) and racemic trans -CHDA (1.14 mg, 0.01 mmol) was combined and dissolved in CDCl 3 (2 mL). The corresponding reaction mixture was heated at 50 °C for 6 h. A [2 + 4] achiral cage ( 2 2 R 2 S 2 , 3 2 R 2 S 2 or 4 2 R 2 S 2 ) was self-assembled as the major product in the 1 H NMR spectrum, without further manipulation. The solid-state sample of each cage was obtained by adding MeOH into its solution in chloroform and collecting the precipitate via filtration. However, it is also unsuccessful to purify these cages via precipitation. We thus used NMR yields to quantify the production of 2 2 R 2 S 2 (57 %), 3 2 R 2 S 2 (75 %) and 4 2 R 2 S 2 (71 %), by adding an internal standard in the NMR sample. Self-assembly of 2 2 (EDA) 4 , 3 2 (EDA) 4 and 4 2 (EDA) 4 A 1:2 mixture of the corresponding tetraformyl precursor ( 2, 3 or 4 , 0.005 mmol) and EDA (0.60 mg, 0.01 mmol) was combined and dissolved in CDCl 3 (2 mL). The corresponding reaction mixture was heated at 50 °C for 6 h. A [2 + 4] achiral cage ( 2 2 (EDA) 4 , 3 2 (EDA) 4 or 4 2 (EDA) 4 ) was self-assembled as the major product in the 1 H NMR spectrum, without further manipulation. The NMR yield of 2 2 (EDA) 4 , 3 2 (EDA) 4 and 4 2 (EDA) 4 was determined to be 50%, 85% and 77%, respectively. Self-assembly of 3 3 S 6 A 1:2 mixture of 3 (3.63 mg, 0.005 mmol) and ( S,S )-CHDA (1.14 mg, 0.01 mmol) was combined and dissolved in CDCl 3 (2 mL). The corresponding reaction mixture was heated at 50 °C for 12 h. 3 3 S 6 was self-assembled as the major product in the corresponding 1 H NMR spectrum, without further manipulation. The NMR yield of 3 3 S 6 was determined to be 63%. Self-assembly of 0 3 S 6 A 1:2 mixture of 0 (3.13 mg, 0.006 mmol) and ( S,S )-CHDA (1.37 mg, 0.012 mmol) was combined and dissolved in CDCl 3 (2 mL). The corresponding reaction mixture was heated at 50 °C for 24 h. 0 3 S 6 was self-assembled as the major product accompanied with a [2 + 4] product as a kinetic product in the corresponding 1 H NMR spectrum. 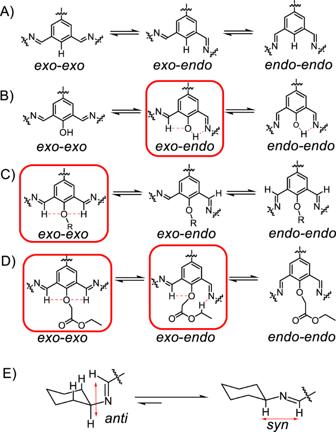Fig. 3: The possible conformations of the imine adducts of isophthalaldehyde derivatives bearing different central substituents between the two imine units. These different central substituents include (A) H, (B) OH, (C) alkoxy (OR) unit, and (D) ester (OCH2COOC2H5) chain. Hydrogen bonding interactions occurs between the central substituents and the two imine units on both sides, which are marked with red dashed lines. OH favors theexo-endoconformation, while the OR unit favorsexo-exoone. In the case of the ester, bothexo-exoandexo-endoare stable conformations, driven by hydrogen bonding with different modes. These relatively stable conformations are encircled with red rectangles. (E) Two conformations of an imine compound, includingsyn(right) andanti(left). Thesynconformer is more favored than theantione due to smaller steric hindrance in the former conformer. As the reaction proceeding, the [2 + 4] kinetic product would transfer to the [3 + 6] chiral cage mostly, but not completely. The NMR yield of 0 3 S 6 was determined to be 70%. General methods Nuclear magnetic resonance (NMR) spectra were recorded at ambient temperature using Bruker AVANCE III 400, Bruker AVANCE III 500, or Agilent DD2 600 spectrometers, with working frequencies of 400/500/600 and 100/125/150 MHz for 1 H and 13 C, respectively. Chemical shifts are reported in ppm relative to the residual internal non deuterated solvent signals (CDCl 3 : δ = 7.26 ppm, DMSO- d 6 : δ = 2.50 ppm). High-resolution mass spectra (HRMS) were measured by using a SHIMADZU liquid chromatograph mass spectrometry ion trap time of flight (LCMS-IT-TOF) instrument and Bruker Daltonics Autoflex III (MALDI-TOF). 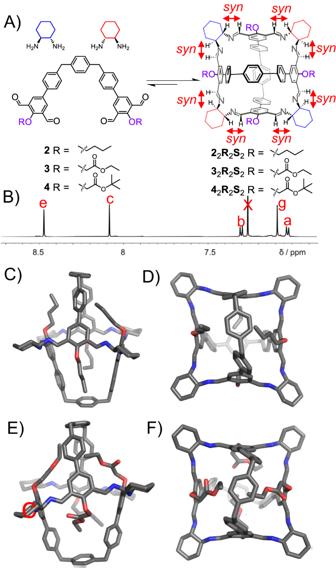Fig. 4: The self-assembly of a series of achiral cages, including 22R2S2, 32R2S2and 42R2S2. (A) Structural formulae of the cages22R2S2,32R2S2and42R2S2, by condensing a 2:1 mixture of racemictrans-CHDA and the corresponding tetraformyl precursor namely2,3and4, respectively. (B) Partial1H NMR spectrum (600 MHz, CDCl3, 298 K) of22R2S2. Some of the key resonances are labeled, which were assigned based on the corresponding two-dimensional NMR spectra shown in the Supplementary Figs.37and38. The full spectrum is shown in the Supplementary Fig.35. Solid-state structures of22R2S2including (C) side view) and (D) top view, as well as32R2S2including (E) side view) and (F) top view, which were obtained from single-crystal X-ray diffraction analysis. Oxygen atoms, red; nitrogen, blue; carbon, gray. Hydrogen atoms and disordered solvent molecules are omitted for clarity. X-ray crystallographic data were collected on a Bruker D8 Venture diffractometer. 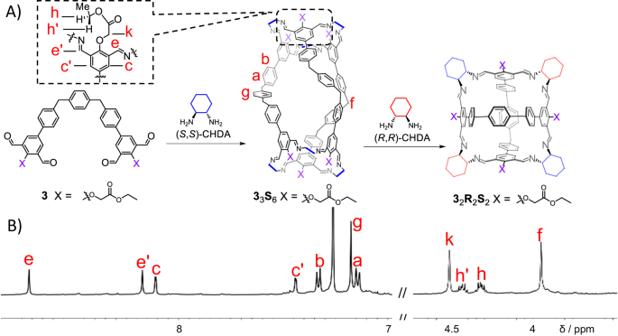Fig. 5: The self-assembly of a chiral cage 33S6that was transformed into 32R2S2upon addition of (R,R)-CHDA. (A) Structural formula of the cage33S6, by condensing a 2:1 mixture of (S,S)-CHDA and3. Upon addition of (R,R)-CHDA,33S6is converted into32R2S2. (B) Partial1H NMR spectrum (600 MHz, CDCl3, 298 K) of33S6. Some of the key resonances are labeled, which were assigned based on the corresponding two-dimensional NMR spectra shown in the Supplementary Figs.60and61. The full spectrum is shown in the Supplementary Fig.58. 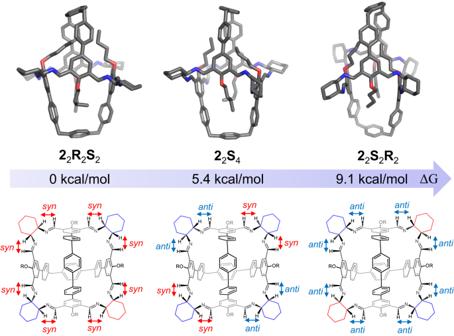Fig. 6: The optimized structures (top) and the structural formula (bottom) of 22R2S2and its two putative less stable counterparts 22S4and 22S2R2, with their corresponding relative free energies. The calculation was performed by using DFT calculations at the level of BP86-D3 functional and 6-311 G(d) basis set. CD spectra were recorded on a Circular Dichroism Spectrometer (Chirascan V100, Applied Photophysics Ltd). Theoretical calculations All investigated cage structures were optimized by using the density functional theory (DFT) at the BP86-D3/6-311G(d) level with the Gaussian 16 package [78] . The solvent effect of chloroform was included with the polarizable continuum model (PCM) [83] . All the optimized structures were verified by the phonon frequencies calculated at the same level (namely no imaginary frequency should exist).